Tip-enhanced photovoltaic effects in bismuth ferrite Photoelectric properties of multiferroic BiFeO 3 , such as large photovoltages exceeding several times the bandgap or switchable photocurrents, have recently generated much interest. This is mostly because of potential applications in photovoltaic or photocatalytic devices. Although the fundamentally different (from classical semiconductors) polarization-related charge separation mechanisms allow unlimited photovoltages, these materials have never been considered a viable alternative to classical semiconductor-based photovoltaics because of a very low light conversion efficiency of less than 10 −4 . Here we investigate the anomalous photovoltaic effect in bismuth ferrite BiFeO 3 single crystals, using photoelectric atomic force microscopy and piezoresponse force microscopy. We show that using a nanoscale top electrode, the photoexcited carriers are efficiently collected and the external quantum efficiency is enhanced by up to seven orders of magnitude. This enhancement might provide a viable alternative for the effective use of the anomalous photovoltaic effect in photovoltaic applications. Bismuth ferrite BiFeO 3 (BFO) is a unique example of an intrinsic multiferroic that simultaneously shows magnetic (antiferromagnetic), ferroelastic and ferroelectric properties at room temperature. Because of its large polarization and its possible coupling with the magnetic moment, BFO is one of the most studied multiferroic materials over the last few years [1] , [2] , [3] , [4] . Recently, the photoelectric properties of BFO have generated much interest [5] , [6] mostly because of its favourable low bandgap of only 2.7 eV, which—unlike other known ferroelectrics such as LiNbO 3 , BaTiO 3 or Pb(Zr,Ti)O 3 —is in the visible range. Anomalously large photoexcited voltages that exceed several times the bandgap have been recently reported on BFO thin films [7] . This effect, including the photogalvanic effect [8] , [9] , makes BFO attractive for applications in photovoltaic or photocatalytic devices [10] . However, a major limitation in using these photoelectric effects in real applications is the extremely low power conversion efficiency, which is in the range of 10 −4 or less [6] , [9] , [11] . Here we investigate the anomalous photovoltaic effect in BFO single crystals by using photoelectric atomic force microscopy (PhAFM) combined with piezoresponse force microscopy (PFM). Here we show that the non-equilibrium photoexcited carriers are uniformly generated over the entire crystal and do not massively recombine within the ferroelastic domains. We also show, besides a high-resolution analysis of the local distribution of photovoltage and photocurrent, that the atomic force microscope (AFM) tip enables an effective collection of the photogenerated non-equilibrium carriers, thus enhancing the external quantum efficiency (QE) by up to seven orders of magnitude. This nanoscale enhancement opens a viable alternative for the effective use of the anomalous photovoltaic effect in photoelectric applications. Bulk photovoltage BFO single crystals that are (100)-oriented were grown using a method similar to that proposed by Kubel and Schmid [12] . Details on growth and sample preparation are given in the Methods section and in Supplementary Methods . For the sake of simplicity throughout the present paper, the pseudocubic crystallographic indexing is used to show the crystallographic orientation of the BFO crystals and the scan directions. Bulk photovoltage and photocurrent measurements were recorded on capacitor-like structures, as well as on crystals that were sideways contacted (see Supplementary Fig. S1 ). 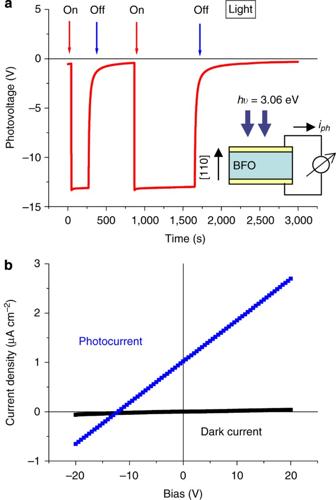Figure 1: Bulk photovoltage properties of BFO. (a) Photovoltage measured on a capacitor structure with a (110)-oriented BFO crystal sandwiched between two Pt electrodes. The inset shows the measurement setup schematically; (b) photocurrent–voltage characteristics in the dark and under illumination. Illumination was performed by an 80-mW violet laser (λ=405 nm) through the semitransparent top electrode. BFO, bismuth ferrite BiFeO3. Figure 1a shows the open-circuit photovoltage measured on a (110)-oriented BFO single crystal by illumination with a 405-nm ( hν= 3.06 eV) laser. The open-circuit photovoltage is ~13 V, equivalent to a field of ~2.6 kV cm −1 , but depending on the crystal it can vary from 6 V to more than 30 V. The photocurrent density is ~1 μA cm −2 ( Fig. 1b ). Figure 1: Bulk photovoltage properties of BFO. ( a ) Photovoltage measured on a capacitor structure with a (110)-oriented BFO crystal sandwiched between two Pt electrodes. The inset shows the measurement setup schematically; ( b ) photocurrent–voltage characteristics in the dark and under illumination. Illumination was performed by an 80-mW violet laser ( λ =405 nm) through the semitransparent top electrode. BFO, bismuth ferrite BiFeO 3 . Full size image Photoelectric atomic force microscope It has been recently proposed that the domain walls have a major role in generating the large photovoltage in BFO [7] . To verify this role, a method is required that allows the mapping of the photoelectric signal with a resolution close to the domain wall width, that is, 1–2 nm. For this purpose, we have developed an AFM-based measurement of the local photoelectric effect, namely PhAFM, which is able to map the photogenerated currents with a lateral resolution in the same order of magnitude as the tip contact diameter, that is, ~20 nm. The setup described in Supplementary Figure S2 consists of an AFM modified by a homemade current-amplifying circuit and an optical system that is able to illuminate the sample surface and map the generated photocurrents. The photoexcitation is performed by a laser with the photon energy of 3.06 eV ( λ =405 nm), which is larger than the BFO bandgap of ~2.7 eV. In this way, the expected optically induced transitions in BFO are of band-to-band type, respectively, from the valence band to the conduction band. With the help of a switching system, one can switch the AFM between the PFM mode and the PhAFM mode, allowing imaging of both ferroelectric domains and the surface distribution of the photocurrent of the same area. Thus, a direct correlation between the ferroelectric domains and/or domain walls and the photoelectric signal is rather straightforward. Nanoscale photovoltaic measurements The first screening of the optically polished surface, using PFM revealed that the BFO crystals exhibit a rich domain pattern, which consists of large-area single domains mixed with areas of smaller periodic domains. The domain pattern, as revealed by the contrast in the phase image of both out-of-plane and in-plane PFM, comprises mostly 109° domains, according to the analysis conducted by Zavaliche et al . [13] The optically polished surfaces exhibit shallow scratches, only 2- to 5-nm deep, which proved to be very detrimental for the photogenerated currents (see Supplementary Fig. S3 ). Scratches and all other mechanical surface defects function as recombination centres and hide most of the intrinsic features of the photocurrent that might be related to the ferroelectric domains. We found that a further chemical–mechanical polishing (CMP) of the crystal not only significantly improves the surface quality but also reveals the ferroelectric domain pattern in the topography. 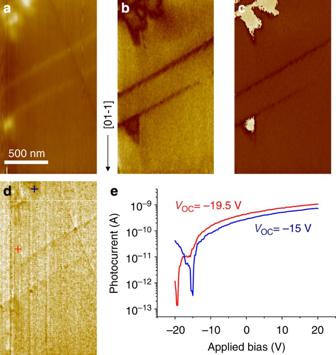Figure 2: PFM and PhAFM on a (100)-oriented BFO single crystal. Topography (a), out-of-plane PFM amplitude signal (b) and phase (c), and the corresponding PhAFM signal (d). Local photoelectric current–voltage characteristics and correspondingVocare shown in (e) for the points marked in (d). The scan direction (shown by an arrow) is along the 01-1 crystallographic direction; the orientation of polarization at the surface is shown inSupplementary Methods. BFO, bismuth ferrite BiFeO3; PFM, piezoresponse force microscopy; PhAFM, photoelectric atomic force microscopy. Figure 2 and Supplementary Figure S4 show a typical domain pattern in an area with a large domain, as revealed by PFM, and the corresponding photocurrent signals. The photocurrent is generated over the whole scanned area and shows a pattern quite similar to the pattern of the PFM amplitude signal. The photocurrent is essentially constant across the entire scanned area, the contrast in the PhAFM image being generated mostly by a 15–20% decrease of the photocurrent in the regions with polarization pointing upwards or at the domain boundaries. This shows that the non-equilibrium photoexcited carriers do not recombine massively within the bulk of the ferroelectric domain, as assumed by Yang et al . [7] Figure 2: PFM and PhAFM on a (100)-oriented BFO single crystal. Topography ( a ), out-of-plane PFM amplitude signal ( b ) and phase ( c ), and the corresponding PhAFM signal ( d ). Local photoelectric current–voltage characteristics and corresponding V oc are shown in ( e ) for the points marked in ( d ). The scan direction (shown by an arrow) is along the 01-1 crystallographic direction; the orientation of polarization at the surface is shown in Supplementary Methods . BFO, bismuth ferrite BiFeO 3 ; PFM, piezoresponse force microscopy; PhAFM, photoelectric atomic force microscopy. Full size image Open-circuit voltages and local photocurrent The open-circuit voltage ( V oc ), determined as the voltage at which the current becomes zero, can be as large as 30 V. V oc varies on the sample surface as well as from sample to sample from about 5 V to more than 40 V. Despite this, a correlation between the macroscopic and nanoscale measurements could be easily carried out by recording both macroscopic and nanoscale measurements under the same illumination conditions. 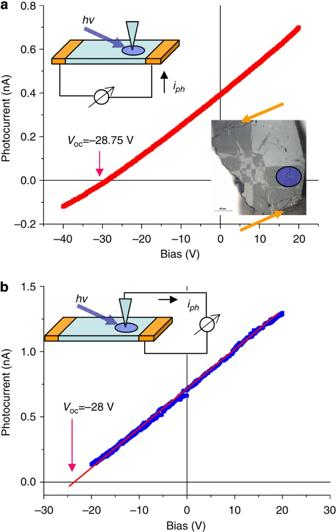Figure 3: Photocurrent–voltage characteristics. (a) Measured macroscopically across the entire crystal by illumination in the region marked in the lower right inset, and (b) measured by probing with the AFM tip in the middle of the illuminated area. The upper left inset in (a) schematically shows the measurement setup and the connection to the macroscopic measurement; the lower right inset in (a) shows the crystal with silver electrodes marked by arrows and approximately the illuminated area by the laser spot. The inset in (b) shows the measurement setup for the local measurements by the AFM tip. The area of this specific measurement and details of the crystallographic orientation are given inSupplementary Figure S1. AFM, atomic force microscopy. Figure 3 shows photoelectric current–voltage characteristics acquired both macroscopically and nanoscopically on the same illuminated area. Figure 3: Photocurrent–voltage characteristics. ( a ) Measured macroscopically across the entire crystal by illumination in the region marked in the lower right inset, and ( b ) measured by probing with the AFM tip in the middle of the illuminated area. The upper left inset in ( a ) schematically shows the measurement setup and the connection to the macroscopic measurement; the lower right inset in ( a ) shows the crystal with silver electrodes marked by arrows and approximately the illuminated area by the laser spot. The inset in ( b ) shows the measurement setup for the local measurements by the AFM tip. The area of this specific measurement and details of the crystallographic orientation are given in Supplementary Figure S1 . AFM, atomic force microscopy. Full size image The local and macroscopic values of V oc correlate very well, but strikingly the absolute value of the current measured between the lateral electrodes on the bulk crystal and at nanoscale through the AFM tip are almost the same. In this specific case, the nanoscale current is higher, but as a rule the nanoscale current is of the same order of magnitude as the current measured macroscopically. This means that the AFM tip collects the same amount of non-equilibrium carriers as do the lateral electrodes. The current density in the macroscopic case is ~4×10 −7 A cm −2 , whereas through the AFM tip the current density can be from 10 to 100 A cm −2 , depending on the effective contact area. This increase by about eight orders of magnitude in the current density leads to the conclusion that the AFM tip is, on one side, very efficient in collecting the photoexcited carriers and, on the other side, that the QE of this effect is rather high. A simple estimation (see Supplementary Methods ) of the external QE at the given wavelength yields for the macroscopic measurements a value of ~3×10 −7 and for the nanoscale measurement a value of ~1.0, which indeed represents an enhancement by seven orders of magnitude. This large QE, sometimes larger than unity, in this case can be understood as a tip enhancement. It is due to the particular geometry of the top electrode, a point-contact geometry with nanoscale dimensions. This geometry has a twofold effect on the photoelectric current. First, the local electric field, which might be considered as produced by the open-circuit photovoltage applied through the tip, is not anymore a uniform field. Actually, it is drastically enhanced at the crystal surface below the tip and strongly confined there, as in the case of other AFM-based measurements such as PFM [14] , [15] . The field lines expand roughly radially in all directions and the isopotential lines describe a slightly prolate semispheroid, most of the field being confined in this volume under the tip. This non-uniform field results in the effective volume from which the photoexcited carriers will drift to the electrode (tip) to be significantly larger than the tip-surface contact area, unlike in the case of a parallel field (macroscopic case). The effective area from which the carriers are collected can be estimated by considering the effective field distribution under the tip. As we have here a transport phenomenon of non-equilibrium carriers in a strong confined field, we would rather prefer not to use the electrostatic models, such as the one proposed by Kalinin et al . [14] for PFM, but instead use models related to charge transport. We consider that the space charge limited conduction mechanism and a point-contact geometry are a good approximation of our case [16] . This assumption is based on previous observations of a space charge limited conduction mechanism in BFO films [17] and is also due to the particular point-contact geometry of the AFM tip. As shown schematically in Supplementary Figure S5 , and considering the analysis presented in the Supplementary Methods , the electric field will decay from the point contact with 1/r 2 , where r is the spherical coordinate pointing from the top electrode into the bulk (BFO crystal). If we assume that the carriers will be effectively collected from a distance at which the field will decay ten times its value under the tip, we obtain an effective radius of about three times the tip-surface contact radius. This means that the effective illuminated area that generates the photocurrent is about ten times larger than the tip-surface contact area, namely the electric contact. Bearing this in mind, the internal QE can be obtained by renormalizing the effective QE to this effective area. Thus, the internal QE ranges from ~0.1 to ~0.4. Even so, this internal QE represents a rather high value for an anomalous photovoltaic and/or a photogalvanic effect. To understand this enhancement in QE by several orders of magnitude, we need to consider where the non-equilibrium carriers are generated. As the photon energy is slightly above the bandgap, the light is absorbed in a shallow region under the surface. According to the Beer-Lambert law the light intensity decays exponentially into the material as I ( x )= I 0 exp (− αx ), where I(x) is the intensity at the distance x into the material, I 0 the light intensity at the surface and α the absorption coefficient. The penetration depth defined as the distance from the surface at which the light intensity decays e times is in this case about 50 nm, considering an absorption coefficient of ~0.018 nm −1 (ref. 18 ). This value is close to the distance at which most of the effective field drops, in other words, the penetration depth of the light is almost the same as the characteristic dimension of the field confinement. This might compensate the low mobility of the carriers and increase the collection efficiency. The main advantage of the abnormal photovoltaic effect is the open-circuit voltage V oc that is not limited by the bandgap, as in the case of semiconductor junctions; it can have any value. In turn, the absolute values of the photocurrents are very small. The present nanoscale enhancement would be really useful in potential applications if it would be scalable with the number of tips. To show this, we have used AFM chips provided with three cantilevers and have measured the photocurrent by successively contacting each tip. 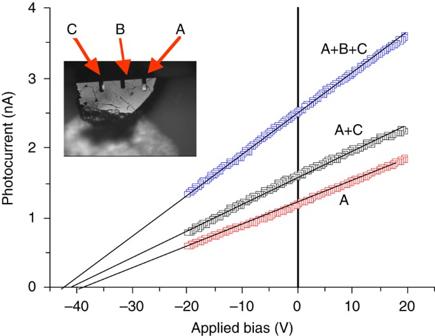Figure 4: Photocurrent upscaling. Photocurrent–voltage characteristics obtained by successively contacting three tips of a multicantilever AFM chip. The lines represent a linear fit to extrapolate theI–Vcharacteristic toVoc. The three cantilevers of the same AFM probe chip (NSC 36, μMASCH) have different elastic constants and can be successively brought into contact by moving the AFM stage towards the crystal surface. The tips A and C are at the rim, whereas the tip B is in the middle of the illuminated area. The inset shows an image of the three cantilevers on the (100)-oriented BFO crystal. AFM, atomic force microscopy; BFO, bismuth ferrite BiFeO3. As shown in Figure 4 , the photocurrent increases as the number of contacted tips increases, namely from 1.1 nA for tip A to 1.7 nA for A+B and 2.5 nA for all three tips in contact with BFO. Although the increase in photocurrent does not exactly scale linearly with the number of tips, most probably due to some particular illumination geometry (the outside tips receive less illuminance that the middle tip), the increase is significant and shows the potential upscaling that might be useful for applications. In principle, there is nothing to prevent a parallel connection of a large number of tips and thus increasing the short circuit photocurrent by orders of magnitude. Alternatively, a light concentration due to a resonant plasmon excitation effect might also generate an enhancement in the photovoltaic effect, as in the case of silicon [19] , but this seems to be just a second-order effect. Figure 4: Photocurrent upscaling. Photocurrent–voltage characteristics obtained by successively contacting three tips of a multicantilever AFM chip. The lines represent a linear fit to extrapolate the I – V characteristic to V oc . The three cantilevers of the same AFM probe chip (NSC 36, μMASCH) have different elastic constants and can be successively brought into contact by moving the AFM stage towards the crystal surface. The tips A and C are at the rim, whereas the tip B is in the middle of the illuminated area. The inset shows an image of the three cantilevers on the (100)-oriented BFO crystal. AFM, atomic force microscopy; BFO, bismuth ferrite BiFeO 3 . Full size image In summary, we have shown that the abnormal photovoltaic effect does exist in bulk BiFeO 3 crystals. Using photoelectric AFM, we have shown that the non-equilibrium photoexcited carriers are uniformly generated over the entire crystal and do not massively recombine within the ferroelastic domains. The AFM tip is an effective collector for photoexcited carriers enhancing the photocurrent density and QE by several orders of magnitude in comparison with the bulk effect. The internal QE of the abnormal photovoltaic effect in BFO is similar to that in semiconductor photovoltaic devices and only the high recombination rate of the non-equilibrium carriers within the bulk of the crystal so far prevents real applications of this effect, which might be enabled by the present tip enhancement effect. BiFeO 3 single crystal growth BiFeO 3 (BFO) single crystals were grown using a method similar to the original method proposed by Kubel and Schmid. [12] Depending on the cooling rate, either platelet-like dendritic crystals or rosette-like pyramidal crystals, as described by Burnett et al ., [20] were obtained. All crystals were polished parallel to the surface, which in rosette crystals is the (100)-crystallographic plane. Samples typically larger than 1×1 mm 2 area and 50- to 300-μm thick were obtained. Macroscopic ferroelastic domains were visualized in a polarized light microscope (see Supplementary Fig. S1 ). Sample preparation Optical quality crystal surfaces were obtained by polishing, using 0.25 μm diamond paste. The remaining damaged surface layer and polishing scratches were removed by CMP. CMP was performed usually for 30 min using SiO 2 colloidal solution (Syton) diluted with water in a 1:1 ratio. For bulk photovoltaic measurements, capacitor-like devices were obtained by sputtering of semitransparent (10 nm thick) Pt/Pd (80/20) electrodes on both faces. In-plane measurements, as well as local AFM-based measurements, were recorded on crystals that were sideways contacted by silver paste, which is visible in Supplementary Figure S1(c,d) at the edge of the crystal. Piezoresponse and photoelectric force microscopy Local photoelectric current and domain patterns were mapped using a homemade system based on an AFM (CP-Research, Thermomicroscopes), modified using a homemade current-amplifying circuit shown in Supplementary Figure S2 . The sample area under the conductive AFM tip was illuminated by an 80-mW laser beam of 405-nm wavelength ( hν =3.06 eV) focused into an ellipsoidal spot with an area of ~0.65×0.3 mm. The photogenerated currents are read using a transimpedance amplifier (Femto, DLPCA-200) with an input impedance better than 10 14 Ω and a typical gain of 10 8 . The voltage is further ten times amplified and filtered with a low-pass filter with typical cut-off frequency of 100 Hz and 12 dB. The final output signal is fed into the auxiliary input of the AFM, thus being simultaneously recorded with the topography signal. Using a switching system, the AFM can be switched between the PhAFM mode and PFM mode, thus allowing imaging of both ferroelectric domains and the surface distribution of the photocurrent of the same area. PFM was performed using an ac signal of 2 V amplitude and 11 kHz frequency applied on the AFM tip. Both PhAFM and PFM were performed using the same conductive tip. Several AFM tips with different conductive coatings and elastic constants were used in order to rule out any spurious effects. The used tips were ATEC-EFM (Nanosensors, Pt-coated, 2.5 N m −1 ), NSC 18 (μMasch, Pt- and Au-coated, 3.5 N m −1 ) and NSC 15 (μmasch, Pt-coated and uncoated, 40 N m −1 ). How to cite this article: Alexe, M. & Hesse, D. Tip-enhanced photovoltaic effects in bismuth ferrite. Nat. Commun. 2:256 doi: 10.1038/ncomms1261 (2011).